Unveiling how intramolecular stacking modes of covalently linked dimers dictate photoswitching properties Covalently linked π-stacked dimers represent the most significant platform for elucidating the relationship between molecular alignments and their properties. Here, we present the one-pot synthesis of two intramolecularly π-stacked dimers and disclose how intramolecular stacking modes dictate photoswitching properties. The dimer, which features cofacially stacked chromophores and geometrically favours intramolecular photochemical [2 + 2] cycloadditions, displays a nearly irreversible photoswitching behaviour. By contrast, the dimer, bearing crosswise stacked chromophores, is geometrically unfavourable for the cycloaddition and exhibits a highly reversible photoswitching process, in which the homolysis and reformation of carbon−carbon single bonds are involved. Moreover, the chiral carbon centres of both dimers endow these photoswitches with chirality and the separated enantiomers exhibit tuneable chiroptical properties by photoswitching. This work reveals that intramolecular stacking modes significantly influence the photochemical properties of π-stacked dimers and offers a design strategy toward chiral photoswitchable materials. Since the first discovery and subsequent synthesis of [2.2]paracyclophane in the middle of the 20th century [1] , [2] , covalently linked π-stacked dimers have attracted intense research interest, ranging from developing new building blocks and synthetic strategies to investigating chemical consequences of their geometries and through-space electronic couplings between π-conjugated moieties [3] , [4] , [5] , [6] . Among these research focuses, the chemical reactivity arising from molecular geometries is of significant interest to generate novel functional properties. For example, benefited from the well-defined alignments of the two π-moieties, geometrically preferred reactions, such as photo-induced cycloadditions, can be achieved efficiently [7] , [8] , [9] . Another important character of these dimers is their high intramolecular steric repulsion, which may lead to unusually long carbon–carbon single bonds (bond length greater than 1.6 Å) [10] , [11] , [12] . The elongated C−C single bonds are accompanied by the decreasing of bond dissociation energies [13] and thus the increasing of reactivity, for instance, via thermal- or photo-activated bond cleavage [14] , [15] . These remarkable structural features and their accompanying potential photochemical reactivity make covalently linked dimers promising candidates for photo-responsive materials. Nevertheless, the on-demand control over the relative positions of the neighbouring π-moieties of such dimers, although highly important for modulating the properties, remains a challenge. Photoswitchable molecules, which interconvert reversibly between two or more isomers through light irradiation or heat, have received intense attention owing to their wide applications in electronics [16] , [17] , [18] , [19] , photopharmacology [20] , [21] , and molecular machines [22] , [23] . Transferring the chirality into a photoswitch enables the reversible and precise control over chiral information. Many unconventional applications for photoswitches, such as in manipulating supramolecular chirality [24] , [25] , liquid crystalline properties [26] , [27] , [28] , [29] , [30] , and asymmetric catalysis [31] , therefore can be achieved. For instance, Li et al. successfully employed chiral photoswitches as dopants to alter the helical axis of cholesteric liquid crystals [27] . Common photoswitchable building blocks such as azobenzene, diarylethene, and spiropyran, however, do not show chirality or cannot maintain their chirality upon photoswitching. The introduction of stable chirality to them usually requires the additional chiral substituent(s) [27] , [32] , [33] , [34] , [35] or the chiral environment [36] . Herein, we report a one-pot synthesis of cyclopentane-bridged dimeric molecules ( 3a and 3b ) through cascade nucleophilic additions. The intramolecular stacking modes and thus photoswitching properties can be effectively modulated by changing the substituents on the aromatic skeleton. The well-aligned alkene pairs in endo dimer ( 3a ) easily leads to intramolecular photo-induced [2 + 2] cycloaddition, which is nearly irreversible upon UV irradiation at a shorter wavelength. In contrast, the exo dimer ( 3b ) displays outstanding reversible photoswitching properties. The photoisomerization of 3b , undergoing through biradical intermediates, shows excellent fatigue resistance under ambient conditions and large changes in geometries and dipole moments after photoswitching. To our knowledge, incorporating the dimers with different intramolecular stacking modes into photoswitches has never been reported. Furthermore, the chiroptical properties of each enantiomer of 3b can be dramatically modulated by UV irradiation. The enantiopure 3b represents a novel kind of photoswitchable building block bearing chiral characteristics, which is a significant complement to the well-established photoswitches. This work, from the fundamental point of view, provides a deep understanding of the relationship between stacking modes in covalently linked dimers and their photoswitching properties. These results would be important in the future design of photoswitches. Synthesis of covalently linked dimers The synthesis of dimers 3a and 3b was inspired by a serendipitous finding during the preparation of cyclopentadienone 2b (Fig. 1 ), a key synthetic intermediate of corannulene [37] , [38] , [39] . Aldol condensation of 4,7-dimethylacenaphthenequinone ( 1b ) and 3-pentanone produces compound 2b in the presence of KOH in methanol after refluxing for 1 h [40] . An unprecedented dimer 3b based on cyclopentadienone, however, was obtained in 64% yield when the reaction time was elongated to 18 h. Different from the previous work in Diels–Alder (D–A) dimerization of cyclopentadienone [41] , five-membered-ring-bridged dimers are formed in this study due to the presence of KOH, a strong base, in the reaction mixture. To further investigate this reaction, we replaced 1b (R = Me) with acenaphthenequinone ( 1a , R = H) as the starting material. Instead of forming an exo dimer like 3b , an endo -dimer 3a was obtained in 38% yield. The photoisomerization of 3a and 3b is also displayed in Fig. 1 , which will be discussed in details later. All new compounds were characterized by nuclear magnetic resonance (NMR) and high-resolution mass spectrometry (HRMS). Fig. 1 One-pot synthesis and photochemical reactions of 3a and 3b . Both 3a and 3b are obtained as a pair of enantiomers. The photochemical rearrangements of 3b leading to 4b and 4c are indicated by solid and dashed arrows, respectively. Full size image Single-crystal analysis of the dimers The structures and configurations of 3a and 3b are unambiguously confirmed by single-crystal X-ray analysis (Fig. 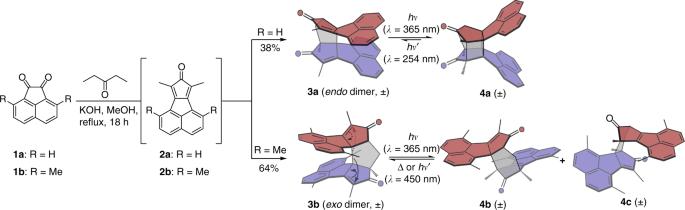Fig. 1 One-pot synthesis and photochemical reactions of3aand3b. Both3aand3bare obtained as a pair of enantiomers. The photochemical rearrangements of3bleading to4band4care indicated by solid and dashed arrows, respectively. 2 and Supplementary Table 1 ). The single-crystal structures of 4a and 4b are also shown here, which will be discussed later. A pair of enantiomers are observed for both 3a and 3b in single crystals (Supplementary Fig. 1 ). In dimers 3a and 3b , two conjugated monomers are bridged by a five-membered ring. In dimer 3a , the monomers are aligned on the same side of the bridge, hence giving an endo configuration. From the top view of 3a , two chromophores containing alkene moieties are nearly cofacially aligned. 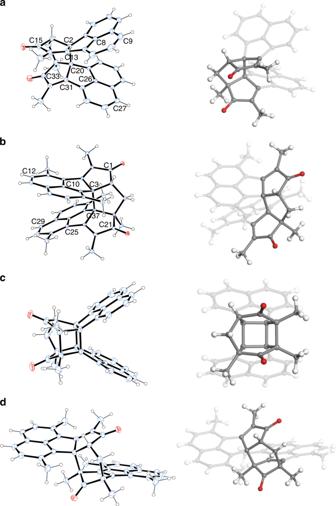Fig. 2 Single-crystal structures.a3a,b3b,c4a, andd4b. Thermal displacement ellipsoids are shown at the 25% probability level. The annulated rings are highlighted. The stacking angle ( θ ), as defined in Supplementary Table 2 , was determined as 11.4°. The distances between two intramolecular stacked arms are ranging from 2.67 to 5.29 Å (Supplementary Table 2 ). Arising from the steric hindrance between two chromophores, the length of the bond connecting two chromophores (C2–C20 single bond) is 1.66 Å, much larger than the typical length for a carbon–carbon single bond (1.54 Å) [42] . Dimer 3b exhibits an exo configuration with the two chromophores stacked crosswise. The stacking angle ( θ ) is determined as 102.8°, much larger than that of 3a (Fig. 2b ). The distances between face-to-face benzenes are ranging from 3.31 to 4.45 Å (Supplementary Table 2 ). The C3–C37 single bond exhibits a length of 1.62 Å, which is also larger than the typical length of carbon–carbon single bond. Fig. 2 Single-crystal structures. a 3a , b 3b , c 4a , and d 4b . Thermal displacement ellipsoids are shown at the 25% probability level. The annulated rings are highlighted. Full size image Mechanism of dimerization To give insights into the reaction mechanism of the dimerization process, a cascade process of nucleophilic additions is proposed (Fig. 3 ). The mechanism for the formation of 3a is illustrated in Fig. 3a ( 3b was formed in a similar process but with a different stereoselectivity). The proposed mechanism can be roughly divided into three stages. The first stage is an Aldol condensation between 1a and 3-pentanone, producing the dehydrated product 2a . This reaction has been thoroughly investigated, and 2a can be separated out [40] . The second stage is a nucleophilic addition between two cyclopentadienonyl derivatives ( 2a ) after one of them is deprotonated on the β -carbon of its carbonyl group. In this step, two out of four chiral centres are determined, and the linkage between monomers is formed, producing enolates 7 . In the third step, a Michael addition takes place, thus presenting the final configuration. Fig. 3 Proposed mechanism. a Proposed mechanism of the nucleophilic addition cascade process. Free energy profiles of Path-endo (black) and Path-exo (blue) for the dimerization of b reactant 2a and c reactant 2b . Values (in kcal·mol −1 ) represent the relative free energies calculated by the ωB97X-D//M11 method in methanol. The values in parentheses are the relative enthalpy. Full size image To elucidate the origin of stereoselectivities during the formation of 3a and 3b , density functional theory (DFT) calculations were employed. Taking 3a for example, two competitive pathways leading to 3a or 3a - exo are considered and the free energy profiles are summarized in Fig. 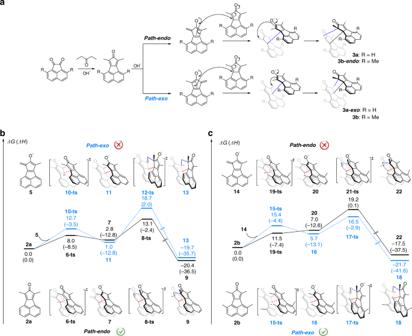Fig. 3 Proposed mechanism.aProposed mechanism of the nucleophilic addition cascade process. Free energy profiles ofPath-endo(black) andPath-exo(blue) for the dimerization ofbreactant2aandcreactant2b. Values (in kcal·mol−1) represent the relative free energies calculated by the ωB97X-D//M11 method in methanol. The values in parentheses are the relative enthalpy. 3b and Supplementary Table 3 . The total free energy of cyclopentadienonyl 2a and its conjugate base 5 (which could be generated by deprotonation of 2a in the presence of base) is set as the relative zero in the free energy profiles. In the Path-endo , the initial intermolecular nucleophilic addition of 5 to the benzyl position on 2a via transition state 6-ts generates enolate complex 7 with a free energy barrier of 8.0 kcal·mol −1 . The subsequent intramolecular cyclization leads to the formation of intermediate 9 , from which the endo dimeric product 3a can be generated after protonation. The overall activation free energy of Path-endo was calculated as 13.1 kcal·mol −1 . Alternatively, the isomer 3a- exo can also be generated in a similar way ( Path-exo ). The corresponding activation free energy of this process (via 12-ts ) was calculated to be 18.7 kcal·mol −1 , much higher than that of Path-endo (via 8-ts ), indicating that the generation of 3a in the endo configuration is more favourable. Non-covalent interaction (NCI) analysis [43] reveals that the energetic discrepancy is mainly contributed by intramolecular π–π interactions between two fragments lowering the energy of transition state 8-ts (Supplementary Fig. 2 ). However, when methyl groups are introduced on naphthalene in the case of 3b , the steric hindrance of methyl groups results in a high activation free energy of 19.2 kcal·mol −1 in Path-endo , which is higher than that in Path-exo (16.5 kcal·mol −1 , Fig. 3c ), leading to the preferable formation of 3b in the exo configuration. These theoretical calculations confirm that both π-π interactions and steric hindrance play important roles in the stereoselectivity of this reaction and illustrate that how the small changes of substituents (H vs. Me) afford completely different configurations. Photoswitching properties of the dimers Initial insights into the photochemical behaviours of cyclopentadione dimers produced by D–A reactions in 1980s [41] , [44] , [45] inspired us to investigate the photoswitching properties of the two obtained dimers. The photoisomerization results of 3a and 3b is shown in Fig. 1 . The parallel alkene pairs in 3a geometrically favour the photochemical [2 + 2] cycloaddition to produce 4a . The intramolecular cycloaddition reaction of 3a in CHCl 3 was monitored by in-situ UV-vis absorption spectroscopy, which indicates that the reaction finishes in less than 16 s upon UV irradiation at 365 nm (Supplementary Fig. 3 ). The quantitative conversion from 3a to 4a was demonstrated by in-situ 1 H NMR spectroscopy (Supplementary Fig. 4 ). The cycloaddition reaction can even happen in single crystals, which was confirmed by in-situ single-crystal X-ray diffraction of 3a before and after UV irradiation. The cycloaddition is irreversible upon heating at 50 °C and nearly irreversible upon UV irradiation at a shorter wavelength ( λ = 254 nm). Upon UV irradiation at 254 nm for 9.5 h, less than 4% of 4a undergoes photocleavage of the cyclobutane to recover to 3a (Supplementary Fig. 4 ). Nonetheless, the four chiral centres on 3a endow its enantiopure forms, i.e. RSSS- 3a and SRRR- 3a (Supplementary Fig. 1 ), with tuneable chiroptical properties upon UV irradiation (Supplementary Fig. 12a and Fig. 12b ). Dimer 3b , however, exhibits completely different photoisomerization behaviours. Two new sets of signals appeared in 1 H NMR upon UV irradiation at 365 nm (Fig. 4b ). This photoisomerization is reversible upon heating. After being heated at 40 °C for 8 h, the mixture completely changed to the initial state (Fig. 4c ). The photoisomerization products of 3b can be separated out from the starting material by column chromatography over silica gel. A yellow solid containing two compounds (i.e. 4b and 4c , which cannot be separated due to their similar polarities and thus are characterized as a mixture) was obtained. The [ 4b ]:[ 4c ] ratio is around 4.1: 1 (determined from the integrations of the peaks at 7.77–7.78 ppm for 4b and at 7.79–7.80 ppm for 4c in 1 H NMR spectra). The structure of the main portion 4b was determined by single-crystal X-ray analysis (Fig. 2d ). One of the arms of 4b isomerizes to an acenaphthylene derivative and its relative orientation to the other arm is also changed. σ[l,3] shifts were first considered as the possible mechanism of the isomerization, but it should be noted that the thermal [1,3] shifts proceeding through suprafacial shifts are forbidden [46] . We therefore proposed a biradical mechanism to explain this isomerization (Fig. 5 ). Upon UV irradiation, the overlong C3−C37 single bond (Fig. 2 ), resulting from the steric repulsion between two cyclopentadienone derivatives, is broken to form biradical intermediate A , which has two resonant structures B and C . The biradicals of B and C form new carbon−carbon single bonds to produce 4b and 4c , respectively. The 1 H NMR spectrum of the less portion is in accordance with the structure of 4c (Supplementary Fig. 5 ), which confirms the proposed mechanism. This homolytic bond breaking and formation mechanism is also found in imidazole-based photoswitches [47] , [48] . DFT calculations reveal that the energy of 4b is about 1 kcal·mol −1 (ωB97X-D/6-31 G(d,p) in the gas phase) lower than that of 4c , which accounts for the larger population of 4b than that of 4c in the photostationary state (PSS). The conversion percentage from 3b to 4b and 4c in the PSS determined by high-performance liquid chromatography (HPLC) is 93% (Supplementary Fig. 6 ), in agreement with the 1 H NMR result (90%). The similar isomerization via biradical intermediates was not observed for 3a , although the length of C2−C20 bond for 3a is 1.66 Å, probably because the rate of photo-induced cycloaddition is much faster than that of the isomerization through biradical intermediates. Fig. 4 Photo- and thermal-isomerization monitored by NMR. 1 H NMR spectra of 3b a in the pristine state, b in the photostationary state ([ 4b + 4c ]/[ 3b ] = 90/10 from the integrations of the peaks at 7.77−7.80 ppm and 6.78−6.79 ppm) and c in the recovered state after being heated at 40 °C for 8 h in CD 2 Cl 2 (4.6 mM). Full size image Fig. 5 Proposed biradical mechanism of the photoswitching process of 3b . The photoisomerization from 3b to 4b was shown in Supplementary Movie 1 . Full size image This photoisomerization results in large difference in geometries and dipole moments between 3b and its photoisomers. 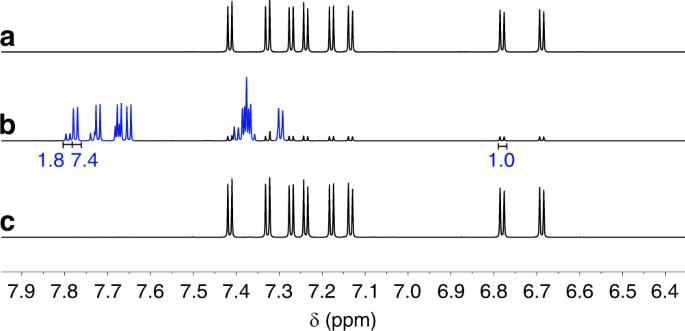Fig. 4 Photo- and thermal-isomerization monitored by NMR.1H NMR spectra of3bain the pristine state,bin the photostationary state ([4b+4c]/[3b] = 90/10 from the integrations of the peaks at 7.77−7.80 ppm and 6.78−6.79 ppm) andcin the recovered state after being heated at 40 °C for 8 h in CD2Cl2(4.6 mM). Compounds 4b and 4c show similar dipole moments, geometries, and absorption (Supplementary Table 4 and Supplementary Fig. 7 ). Therefore, even though they cannot be easily separated, they can still be regarded as one portion when they are used as a photoswitch. Herein, the main portion 4b is used as an example to illustrate the difference from 3b . The end-to-end distances are increased from 4.7 Å for 3b to 8.8 Å for 4b (Supplementary Table 4 ), generating a difference of 4.1 Å in length, which is larger than that of the E/Z isomerization of azobenzene (~3.5 Å [17] ). This large geometrical change in chemical structures is expected to induce significant morphological difference in hierarchical assemblies and thus provides the possibilities in the control of protein folding and unfolding [49] , artificial molecular muscles [50] and supramolecular chemistry [51] . In addition, the dipole moments change from 6.2 Debye for 3b to 2.7 Debye for 4b due to the shift of relative orientations of two arms. To reveal kinetic processes of the thermal isomerization from 4b and 4c to 3b , time-dependent 1 H NMR spectra of the solution of 3b in the PSS at various temperatures were measured. The thermal isomerizations of 4b and 4c follow first-order kinetics (Supplementary Fig. 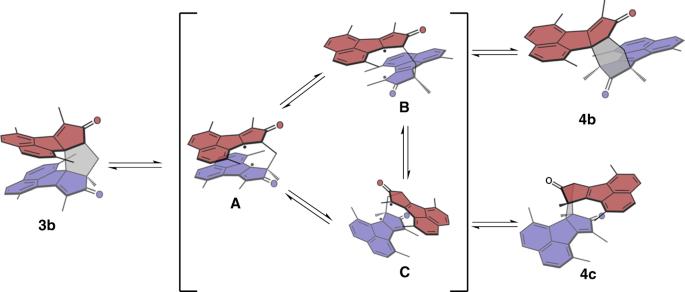Fig. 5 Proposed biradical mechanism of the photoswitching process of3b. The photoisomerization from3bto4bwas shown in Supplementary Movie1. 8 and Supplementary Table 5 ). At room temperature (298 K), the activation energy of the thermal isomerization from 4b to 3b was determined to be 24.8 kcal·mol −1 with a half-life of 3.87 h and that from 4c to 3b was 24.5 kcal·mol −1 with a half-life of 4.05 h. The photoswitching process of 3b was also monitored by UV-vis spectroscopy (Fig. 6a-c ). Three isobestic points at 300 nm, 371 nm and 406 nm are observed upon UV irradiation at 365 nm. The absorbance from 300 nm to 369 nm and from 406 nm to 500 nm increases as the UV irradiation time extends. The onset absorbance red-shifts from 428 to 500 nm. The photoisomerizations reach the PSS in less than 70 s. After being heated at 55 °C for less than 45 min, the mixture recovers to pristine state entirely. To test the photostability of 3b , 4b , and 4c , the solution of 3b was alternately irradiated with UV light and heated, and the absorbance at 343 nm was selected to monitor the photoswitching process. The switch exhibits no fatigue after 10 repeated cycles under ambient conditions (Fig. 6c , temperature: ~28 °C, humidity: 75–90%), indicating a large fatigue resistance of the photoswitching process. 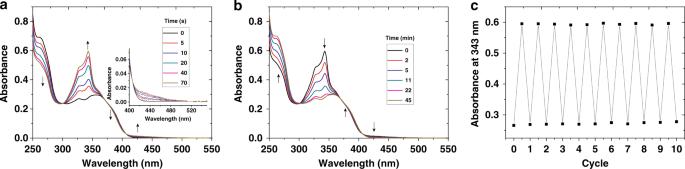Fig. 6 Photo- and thermal-isomerization monitored by absorption spectra. Absorption of3baupon UV irradiation 365 nm andbthen heated at 55 °C (CHCl3, 2.24 × 10-5M);cabsorbance at 343 nm upon UV irradiation at 365 nm for 70 s and then heated at 55 °C for 45 min in repeated cycles. 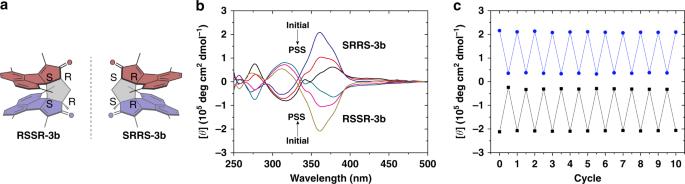Fig. 7 Chiral photoswitching of3b.aEnantiomers of3b.bCD spectra of RSSR-3band SRRS-3bupon UV irradiation at 365 nm.cMolar ellipticity at 360 nm upon UV irradiation at 365 nm for 70 s and then heated at 55 °C for 45 min in repeated cycles (SRRS-3bin blue line and RSSR-3bin black line). To confirm if the thermal-back isomerization can be achieved by light irradiation, the PSS solution of 3b was irradiated with visible light at 450 nm. The back isomerization from 4b and 4c to 3b is indeed accelerated (Supplementary Fig. 9 ), revealing the photoisomerization of 3b is reversible both upon heating and light irradiation. Fig. 6 Photo- and thermal-isomerization monitored by absorption spectra. Absorption of 3b a upon UV irradiation 365 nm and b then heated at 55 °C (CHCl 3 , 2.24 × 10 -5 M); c absorbance at 343 nm upon UV irradiation at 365 nm for 70 s and then heated at 55 °C for 45 min in repeated cycles. Full size image The enantiomers of 3b (RSSR- 3b and SRRS- 3b ) can be separated by chiral HPLC (Supplementary Fig. 10b ). Comparison of their circular dichroism (CD) spectra and the corresponding DFT-simulated ones reveals that the component eluting at 13.6 min is RSSR- 3b , and that eluting at 15.7 min is RSSR- 3b (Supplementary Fig. 11b ). As expected, RSSR- 3b and SRRS- 3b show mirror-like CD spectra (Fig. 7b ). The chiroptical properties of RSSR- 3b and SRRS- 3b can be altered by UV irradiation at 365 nm. For example, the exciton couplet of SRRS -3b at 360 nm weakens as the irradiation time increases and fully recovers after being heated at 55 °C for 45 min (Supplementary Figs. 12c and 12d ). The molar ellipticity of SRRS -3b at 360 nm is switched from 2.1 × 10 5 (ON state) to 3.7 × 10 4 deg·cm 2 ·dmol -1 (OFF state) with a ON/OFF ratio at 5.7 upon UV irradiation. The chiral properties exhibit no decay after ten repeated switching cycles (Fig. 7c ). Such high fatigue resistance under ambient conditions outperforms that of most reported chiral photoswitches [32] , [35] , [47] . These outstanding properties make the chiral photoswitches highly promising building blocks for the applications in modulating supramolecular chirality, chiral information storage, asymmetric synthesis, etc. Fig. 7 Chiral photoswitching of 3b . a Enantiomers of 3b . b CD spectra of RSSR- 3b and SRRS- 3b upon UV irradiation at 365 nm. c Molar ellipticity at 360 nm upon UV irradiation at 365 nm for 70 s and then heated at 55 °C for 45 min in repeated cycles (SRRS- 3b in blue line and RSSR- 3b in black line). Full size image In summary, a new type of cyclopentane-bridged dimeric molecules with different intramolecular stacking modes have been synthesized in a concise one-pot procedure. Their intramolecular stacking modes (i.e. endo or exo configurations) can be modulated by modifying the substituents on the aromatic core, as confirmed by single-crystal structures. Theoretical calculations reveal that such stereoselectivity resulted from the competition between steric repulsion and π–π interactions. The endo -dimer ( 3a ) displays a nearly irreversible photoswitching process through intramolecular photochemical [2 + 2] cycloaddition and its reverse reaction. The exo -dimer ( 3b ) undergoes reversible photoswitching processes via biradical intermediates. This work demonstrates the possibility of tuning intramolecular stacking modes of rigidly linked π-stacked molecules by altering the substituents and provides a chiral photoswitchable building block, i.e. exo -dimer, with excellent properties such as high fatigue resistance and large changes in geometries, chiroptical properties, and dipole moments during photoisomerizations. The exo -dimer is a significant complement to the well-established photoswitches as exemplified by azobenzene, diarylethene, and spiropyran. Further fine-tuning of the photoswitching properties and exploration of their potential applications, for example, in single-molecule electronics [52] , [53] , singlet fissions [54] , [55] , bioimaging [56] , and supramolecular chemistry [49] , [51] , [57] , [58] , require the facile chemical modifications of the exo -dimer. The introduction of reactive groups such as halogens within the precursors may provide photoswitching dimers allowing for versatile late-stage functionalization, which is in progress in our group. Synthesis of 3a A solution of KOH (862 mg, 15.4 mmol) in methanol (10 mL) was added dropwise to a mixture of 1a (350 mg, 1.92 mmol), 3-pentanone (661 mg, 7.68 mmol) and methanol (10 mL) at room temperature. The mixture was stirred at reflux for 18 h. The precipitation was filtered, washed with water and dried under vacuum. The crude product was further purified by column chromatography over neutral alumina (eluent: chloroform/hexane = 3/7) to give 3a (168 mg, 38 %) as a pale-yellow solid. Synthesis of 3b Compound 3b was synthesized using the same methods as described for 3a . It was obtained as a pale-yellow solid (277 mg, 64%). The detailed procedures and characterization are presented in Supplementary Methods . All NMR spectra are shown in Supplementary Figs. 13 – 29 . Single-crystal X-ray diffraction Single-crystal diffraction data were collected on a XtaLAB Synergy, Dualflex, HyPix single-crystal diffractometer using Cu Kα ( λ = 1.54184 Å) micro-focus sealed X-ray tube at 100 K for 3a , 3b and 4a and on a Rigaku SuperNova X-Ray single-crystal diffractometer using Cu Kα ( λ = 1.54184 Å) micro-focus X-ray sources at 150 K for 4b . Computational methods DFT calculations on mechanisms were carried out at the ωB97X-D/6-311 + G (d,p)//M11/6-31 G(d) levels of theory in methanol using a SMD solvation model. DFT calculations on geometries and TD-DFT calculations on optical spectra were performed at the ωB97X-D/6-31 G(d,p) level of theory in the gas phase. The coordinates of all optimized structures are provided in Supplementary Data 1 . Detailed methods are presented in the Supplementary Methods . Kinetic measurements The solution of 3b in CDCl 3 (3.85 mM) was irradiated with UV light ( λ = 365 nm) to the photostationary state and used immediately. The solution of the mixture of 3b , 4b , and 4c was kept at various temperature (303, 308, 313, 318, and 323 K) in dark and characterized by time-dependent 1 H NMR spectra. The temperature was controlled by a water bath. The ambient temperature was around 25 °C. The samples were dipped in ice water for 15 s before the acquisition of 1 H NMR spectra to reduce the decay of the photoisomers resulting from the lingering warmth during the measurements. The concentrations of 3b , 4b , and 4c in the mixture were determined by the integrations of the peaks with the chemical shifts at 1.19 ppm for 3b , 0.87 ppm for 4b , and 0.77–0.78 ppm for 4c . The initial concentrations were around 2.85 mM for 4b and around 0.61 mM for 4c .